The phase diagram of electron-doped La2−xCexCuO4−δ Superconductivity is a striking example of a quantum phenomenon in which electrons move coherently over macroscopic distances without scattering. The high-temperature superconducting oxides (cuprates) are the most studied class of superconductors, composed of two-dimensional CuO 2 planes separated by other layers that control the electron concentration in the planes. A key unresolved issue in cuprates is the relationship between superconductivity and magnetism. Here we report a sharp phase boundary of static three-dimensional magnetic order in the electron-doped superconductor La 2− x Ce x CuO 4− δ , where small changes in doping or depth from the surface switch the material from superconducting to magnetic. Using low-energy spin-polarized muons, we find that static magnetism disappears close to where superconductivity begins and well below the doping level at which dramatic changes in the transport properties are reported. These results indicate a higher degree of symmetry between the electron and hole-doped cuprates than previously thought. The electron-doped high- T c superconductors are less well-understood than their hole-doped counterparts [1] . Nevertheless, experiments on La 2− x Ce x CuO 4− δ (LCCO), Pr 2− x Ce x CuO 4− δ (PCCO) and Nd 2− x Ce x CuO 4− δ (NCCO) have great significance in the field of condensed matter physics because they provide a way to investigate particle–hole symmetry in the phase diagram where superconductivity emerges from doping a highly correlated antiferromagnetic Mott insulator or charge transfer insulator (see ref. 2 and references therein). In both n - and p -type materials, there appears to be a quantum critical transition as a function of doping, which is characterized by sharp maxima in a variety of properties near absolute zero [3] . Remarkably, the superconducting phases of the hole- and electron-doped materials have the same d -wave pairing symmetry [4] . However, there is uncertainty about the position of the critical doping and even the number of critical points. This results from the difficulty to monitor how the antiferromagnetic phase of the parent compound evolves and changes as a function of doping, especially on the electron-doped side [5] , [6] , [7] . This issue remains of central importance since fluctuations associated with the quantum critical point (QCP) may be the origin of strong superconducting pairing and unusual properties in the normal state [8] , [9] . Although there are many similarities in the generic phase diagrams of hole- and electron-doped cuprates, there are also considerable differences [10] . In particular, the magnetism is much more prominent on the electron-doped side and appears to overlap significantly with superconductivity. Also the superconducting dome is much smaller and narrower in electron-doped systems [2] . Both systems show a pseudogap opening below a temperature T * in the underdoped region, which indicates some kind of fluctuating charge or spin order [6] , [11] , [12] , [13] , [14] . However, it is still unclear whether the character of the pseudogap phase is the same in both the electron- and hole-doped cuprates [2] . As mentioned previously, determining the phase diagram in electron-doped cuprates is complicated by the difficulty in determining how the magnetism evolves and eventually disappears as a function of doping. For example, in NCCO, inelastic magnetic neutron-scattering results show that the long-range antiferromagnetic order disappears close to where superconductivity first appears [6] . However, both Shubnikov-de Haas Oscillations [15] and ARPES measurements [16] find a transition well inside the superconducting dome where the Fermi surface reconstructs. It is unclear what happens in between these two dopings. One possibility is that neutrons detect the disappearance of the long-range three-dimensional (3D) antiferromagnetic order where superconductivity begins. However, another less well-ordered phase persists up to a larger value of x c where the Fermi surface reconstructs, leading to sudden changes in transport properties [17] , [18] . LCCO has very similar properties to PCCO and shows the characteristic T -linear resistivity below a critical doping of 0.17 and Fermi liquid form ( ρ ∝ T 2 ) above [5] . Also recent angular magnetoresistance (AMR) measurements reveal evidence for the disappearance of static magnetism above an optimal doping close to x c =0.14 where many transport properties change abruptly [19] . A major difficulty in determining how the magnetism evolves in La 2− x Ce x CuO 4− δ is that it can only be made in a thin-film form. Therefore, the traditional experimental techniques for studying magnetism such as neutron scattering, NMR and bulk μSR are not applicable. Recently, the technique of low-energy muon spin rotation (LE-μSR) has been developed [20] . In LE-μSR, the mean implantation depth of the muons can be controlled from a few nm to a few hundred nm (see Methods). It is now well established that LE-μSR is a powerful way to investigate both the magnetic and electronic properties of quantum materials [21] , [22] , [23] , [24] . In this paper, we report zero-field (ZF) LE-μSR measurements on thin films of La 2− x Ce x CuO 4− δ with Ce concentrations near the antiferromagnetic-superconducting boundary. The measurements are performed at the μE4 beam-line of the Swiss Muon Source [25] , at the Paul Scherrer Institute, in Switzerland. Samples with Ce concentration of x =0.07, 0.08 and 0.10 were studied and have thicknesses of 200 nm (see Methods). For comparison, a fourth film with a Ce concentration of 0.08 and thickness 100 nm is also studied. Monte Carlo simulations using TRIM.SP [26] , [27] show that the average muon implantation depth in La 2− x Ce x CuO 4− δ ranges from 7 to 110 nm with corresponding straggling of 3 and 23 nm, for implantation energies from 1 to 25 keV, respectively. Both the mean depth and range straggling are close to being linear functions of the implantation energy. Energy dependence of static magnetism Typical ZF-μSR spectra at 5 K and energies 5 and 21 keV in all the films are shown in Fig. 1 . Note that at 21 keV, corresponding to an average implantation depth of d ≈88 nm and range straggling Δ≈20 nm, one can clearly see a fast relaxing signal in the x =0.07 sample (red points in the Fig. 1a ), whereas no such fast component is observable in the two higher dopings at this energy (red points in the Fig. 1b–d ). This demonstrates that there is bulk static magnetism in the x =0.07 film that is absent at the two higher dopings. The behaviour is markedly different at the lower energy of 5 keV, corresponding to d ≈24 nm with Δ≈9 nm (see blue points in Fig. 1 ). In particular, the fast relaxing signal is present in both the 0.07 and both 0.08 samples, but absent in the sample with the x =0.10. The magnetic fraction is slightly larger in the 200 nm thick film compared with the 100 nm film but the transition temperature for the magnetism to disappear is the same (discussed later). It is more subtle but still clear that the signal is less damped at 5 keV compared with 21 keV in the x =0.07 sample (red and blue points in Fig. 1a ). In general, static magnetism is enhanced close to the surface in all four samples, with the contrast being largest in the two x =0.08 samples. 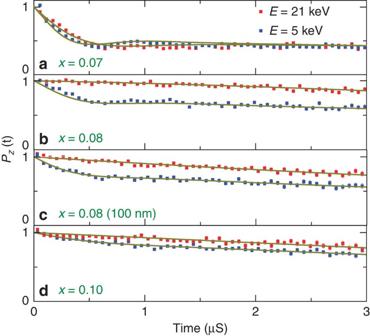Figure 1: Typical ZF-μSR spectra in La2−xCexCuO4−δ. Normalized asymmetry in thin-film samples with Ce concentrations of (a)x=0.07 of thickness 200 nm, (b) 0.08 of thickness 200 nm, (c) 0.08 of thickness 100 nm and (d) 0.1 of thickness 200 nm. All spectra are taken in zero applied magnetic field at a temperature of 5 K. The blue and red points correspond to muon implantation energies of 5 and 21 keV, respectively. The error bars (too small to be seen clearly) indicate one standard deviation. The solid curves are fits described in Methods. Figure 1: Typical ZF-μSR spectra in La 2− x Ce x CuO 4− δ . Normalized asymmetry in thin-film samples with Ce concentrations of ( a ) x =0.07 of thickness 200 nm, ( b ) 0.08 of thickness 200 nm, ( c ) 0.08 of thickness 100 nm and ( d ) 0.1 of thickness 200 nm. All spectra are taken in zero applied magnetic field at a temperature of 5 K. The blue and red points correspond to muon implantation energies of 5 and 21 keV, respectively. The error bars (too small to be seen clearly) indicate one standard deviation. The solid curves are fits described in Methods. Full size image The observed relaxation reported here is due to quasi-static magnetic fields. This was established with longitudinal field measurements where the applied magnetic field is along the initial spin polarization direction. In particular, a longitudinal field of 100 G was enough to quench the observed relaxation in Fig. 1 . This implies the internal magnetic field B must be static on the timescale of muon Larmor frequency γ μ B ≈10 7 s −1 , which is typical of 3D ordering. The energy dependence of the magnetic volume fraction f and average internal field B are shown in Fig. 2 . The x =0.07 sample is fully magnetic at all energies. The internal field is about ~60 G at low energy (near the surface) and decreases only slightly at the higher energy. The x =0.08 sample appears magnetic below ~10 keV, where the mean implantation depth is 40 nm. However, the internal field drops abruptly to zero above 10 keV. The results on the 100 nm thick film with x =0.08 (not shown here) are very similar to the 200 nm thick film indicating these affects are not dependent on the film thickness. In the x =0.1 sample, there is only a very weak magnetic relaxation, which is enhanced slightly close to the surface (see Fig. 1d ). 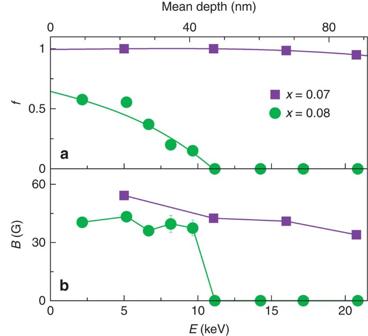Figure 2: Energy dependence of the volume fraction and internal field. (a) Magnetic fractionfand (b) average internal magnetic fieldBas a function of muon implantation energy atT=5 K in LCCO films with Ce concentrationx=0.07 and 0.08. Thexaxis above the top panel shows the corresponding mean implantation depth of low-energy muons in LCCO as simulated by TRIM.SP. Error bars give the fit uncertainties and solid curves are guides to the eye. Figure 2: Energy dependence of the volume fraction and internal field. ( a ) Magnetic fraction f and ( b ) average internal magnetic field B as a function of muon implantation energy at T =5 K in LCCO films with Ce concentration x =0.07 and 0.08. The x axis above the top panel shows the corresponding mean implantation depth of low-energy muons in LCCO as simulated by TRIM.SP. Error bars give the fit uncertainties and solid curves are guides to the eye. Full size image Temperature dependence of static magnetism The maximum magnetic ordering temperature in the region probed by the muons is obtained from the temperature dependence of ZF-μSR spectra, examples of which are shown in Fig. 3 . This shows how the spectrum evolves in the x =0.07 sample going through the magnetic ordering transition. Below the transition, there is a clear evidence for an over-damped oscillation due to quasi-static electronic moments that give rise to a broad distribution of the local internal fields. As one approaches the transition, the magnitude of this average field B drops to zero. Above the transition, in the paramagnetic state, the electronic moments are rapidly fluctuating, so the observed weak time dependence of the muon polarization is due mostly to weak quasi-static nuclear dipolar fields. In the x =0.07 sample at 20 keV (not shown in Fig. 4 ), the fitted magnetic fraction f and the magnitude of the internal field approach zero near 65 K indicating that the entire sample is paramagnetic above this temperature. At 5 keV, much closer to the surface, the transition temperature is much higher (see purple points in Fig. 4 ). In the 0.08 sample, the surface has a magnetic ordering temperature close to 40(5) K (see green points in Fig. 4 ), but the bulk is non-magnetic with no sign of static magnetism. This is evident from the fast relaxing signal at low energies (below 10 keV) as seen earlier in Figs 1 and 2 , compared with the slowly relaxing signal at higher energies. At the highest Ce concentration ( x =0.10), there is no magnetic ordering at any temperature. It is important to note that the muon is sensitive to any static order both short and long range. The absence of any static magnetic field in a μSR experiment (for example, in the x =0.10 sample) implies there is no static 3D magnetism of any type (long-range antiferromagnetism, spin density wave or spin glass). On the other hand, it does not exclude quasi two-dimensional (2D) magnetic order in the planes as long as the internal fields are still fluctuating fast compared with γ μ B ≈10 7 s −1 . 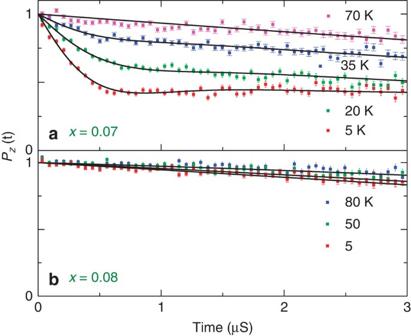Figure 3: Typical ZF-μSR spectra versus temperature. Normalized asymmetry at 21 keV versus temperature in the bulk of La2−xCexCuO4−δfilms with Ce concentrations of (a)x=0.07 and (b) 0.08. Error bars indicate one standard deviation, and the solid curves are fits as described in Methods. Figure 3: Typical ZF-μSR spectra versus temperature. Normalized asymmetry at 21 keV versus temperature in the bulk of La 2− x Ce x CuO 4− δ films with Ce concentrations of ( a ) x =0.07 and ( b ) 0.08. Error bars indicate one standard deviation, and the solid curves are fits as described in Methods. 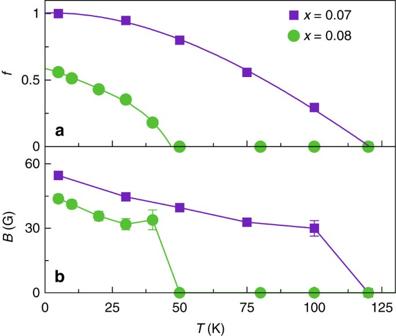Figure 4:T-dependence of the volume fraction and internal field. (a) Temperature dependence of the magnetic fractionfand (b) average internal magnetic fieldB; at 5 keV in LCCO samples with Ce concentrationx=0.07 and 0.08. Error bars give the fit uncertainties and solid curves are guides to the eye. Full size image Figure 4: T -dependence of the volume fraction and internal field. ( a ) Temperature dependence of the magnetic fraction f and ( b ) average internal magnetic field B ; at 5 keV in LCCO samples with Ce concentration x =0.07 and 0.08. Error bars give the fit uncertainties and solid curves are guides to the eye. Full size image Phase diagram The results are summarized in the phase diagram in Fig. 5 . The green circles (5 keV), yellow squares (11 keV) and black diamonds (21 keV) are LE-μSR results for 200 nm thick films. The red and blue triangles are for the 100 nm thick film. The brown band defines the magnetic phase boundary from the LE-μSR measurements, with static magnetism to the left. The width of the band originates from the depth dependence of the magnetism in the film (that is, the phase boundary for the bulk of the film is the left side of the brown band). The dashed blue curve is the superconducting transition temperature obtained from resistivity, while the magenta dashed curve is the magnetic transition temperature obtained from AMR measurements [19] . 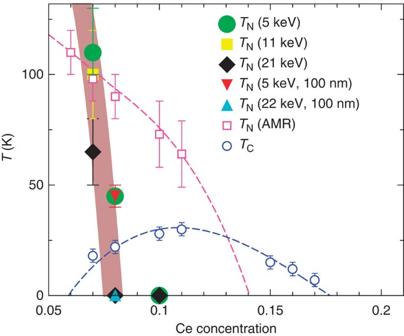Figure 5: An updated phase diagram of LCCO. The magnetic phase boundary measured with LE-μSR is the brown band. The width of the band is due to the depth dependence of magnetism. All data are taken on 200 nm thick films, except one film of 100 nm (triangle symbols). The Néel temperature (TN) from the AMR data is also shown for comparison (from ref.19). Solid and dashed lines are guides to the eye. Error bars of our measurements define the temperature range where magnetism disappears. Figure 5: An updated phase diagram of LCCO. The magnetic phase boundary measured with LE-μSR is the brown band. The width of the band is due to the depth dependence of magnetism. All data are taken on 200 nm thick films, except one film of 100 nm (triangle symbols). The Néel temperature ( T N ) from the AMR data is also shown for comparison (from ref. 19 ). Solid and dashed lines are guides to the eye. Error bars of our measurements define the temperature range where magnetism disappears. Full size image There is a considerable difference in the magnetic phase boundary seen with ZF-μSR and AMR as reported in Fig. 5 . In particular, LE-μSR shows a much narrower region of overlap of the static magnetism with superconductivity. Comparing the results from these two techniques provides an important insight into the nature of the magnetism. AMR and LE-μSR are sensitive to magnetic fluctuations on a much different timescale. As mentioned above, LE-μSR measures the temperature at which the internal fields become static on the scale of the period for the Larmor frequency associated with the internal fields, which in this case is 10 −7 s. On the other hand, the AMR detects magnetism when the fluctuations become much slower than the relaxation time (10 −12 s). Normally this would not shift the ordering temperature very much. However, LCCO is highly anisotropic so that the coupling between moments in the plane is considerably larger than the coupling between planes. Thus, the ordering temperature detected by AMR is determined by the in-plane coupling between spins J . Just below this temperature, the moments are highly correlated in the CuO 2 plane but are still dynamic on the timescale detectable with LE-μSR. The ordering temperature in LE-μSR defines the boundary for static 3D ordering, which depends on and varies logarithmically with the much smaller magnetic coupling between planes J ′ (ref. 28 ). This gives a new insight into the relationship between the magnetism in the region of the SC dome before the Fermi surface reconstructs. Apparently, the moments are still fully developed above T c but are very dynamic on the muon timescale. Finally, we note that the LE-μSR measurements are performed in zero applied magnetic field whereas the AMR measurements are made in a magnetic field of 14 T applied in-plane. It is possible that the large magnetic field used in AMR would frustrate the 2D antiferromagnetic order and thereby suppress ordering temperature [29] . This could explain why the AMR 2D phase boundary seems to cross the LE-μSR 3D phase boundary at x =0.07. From the LE-μSR results in the bulk of the film, we conclude that the 3D static magnetism disappears close to where superconductivity begins and thus there is little overlap region between static 3D magnetism and superconductivity. This is similar to what is found in La 2− x Sr x CuO 4− δ except for the evidence of phase separation in bulk, such that a weak spin glass phase with a small volume fraction extends into the superconducting dome in La 2− x Sr x CuO 4− δ (ref. 30 ). It is possible that a similar spin glass phase exists in LCCO in bulk but the glass temperature would have to be lower than our base temperature of 4 K. Thus, the present results are consistent with a sharp boundary and competition between superconductivity and magnetism without microscopic coexistence. However, comparing these results with AMR leads us to the conclusion that above the SC dome the moments are fully developed and highly correlated within the CuO 2 plane but are still fluctuating without any 3D order. Striking similarities between hole- and electron-doped cuprates are also reported by transport studies [5] . It is now clear there are at least two QCPs in La 2− x Ce x CuO 4− δ . The lower one is near x =0.08 where the antiferromagnetism disappears, whereas the Fermi surface reconstructs at a much higher doping level above x =0.12 (refs 7 , 5 ). It is worth noting that recent studies of certain heavy fermions show a similar phase diagram with two critical points or possibly a line of QCPs called a quantum critical phase in between [31] . The difference in the magnetic behaviour of the surface compared with the bulk of the film is also very interesting. It is possible that small structural changes, expected near a free surface, are enough to tip the balance towards magnetism. This would be consistent with a small difference in (free) energy between competing phases near a critical point. As mentioned previously, LE-μSR measurements were also taken on a thinner (100 nm) sample with x =0.08. The magnetic properties of the free surface were the same as in the 200 nm thick film with the same value of x . However, in the thinner film, it was possible, using 21 keV muons, to probe the interface between the film and the substrate. These measurements showed that this interface was non-magnetic, implying the magnetism is not simply a consequence of the broken translational symmetry and resulting boundary conditions. In conclusion, we have conducted a depth-resolved LE-μSR study of magnetism in La 2− x Ce x CuO 4− δ films close to the magnetic-superconducting transition region. We find that the near-surface region tends to be more magnetic than the bulk of the films. The enhanced magnetism in the near-surface region of x =0.08 is a property of the free surface and absent near the substrate interface. The disappearance of strong static magnetic order in the bulk occurs just below x =0.08, which is close to where superconductivity appears. Above this critical value of x , the moments may exist but are fluctuating rapidly on the muon timescale. The AMR results indicate there is a high degree of 2D order above the superconducting dome. Thus, above the superconducting transition, the system is in a dynamic magnetic state with strong antiferromagnetic correlations. This is similar to the hole-doped counterpart La 2− x Sr x CuO 4− δ and consistent with a competition between order parameters. These results suggest that there may be a higher degree of particle–hole symmetry in this critical region of the phase diagram than previously thought. LE-μSR experiment The measurements are performed using low-energy μSR technique, where an intense high-energy beam of muons is moderated in a solid Ar film. A small percentage of the incident muons emerge from the argon surface at low energy (≈10 eV). These are subsequently accelerated to 15 keV and transported to the sample chamber and μSR spectrometer. The samples are mounted onto a Ag-coated metal plate that is electrically isolated from the cold finger of the cryostat and biased to a high voltage ranging from −12.5 to 12.5 kV. This allows the implantation energy of the muons to be adjusted between about 1.5 and 26.5 keV. The measurements reported here were performed in zero external magnetic field (ZF) such that any stray magnetic field at the sample was less than 0.01 mT. Measurements in a longitudinal field and transverse field were also performed but are not shown here. The time evolution of the muon spin polarization P ( t ), which is measured through the properties of the muon decay, depends on the static and fluctuating components of the internal magnetic field at the site of the muon [32] . Samples The c axis-oriented La 2− x Ce x CuO 4− δ , films were deposited directly on insulating (100) SrTiO 3 substrates by a pulsed laser deposition technique utilizing a KrF excimer laser as the exciting light source. The three films had Ce concentrations of x =0.07, 0.08 and 0.10. Since the oxygen content has an influence on both the superconducting and normal state properties of the material, the annealing process is optimized for each x . We studied three Ce concentration: 0.07 ( T c =18±2 K), 0.08 ( T c =22±2 K) and 0.10 ( T c =27.6±0.5 K). The sample with x =0.1 is metallic (with d ρ /d T >0) above T c with a narrow transition width. The x =0.07 and x =0.08 samples showed an upturn (either in a field or ZF) at low temperature. Each La 2− x Ce x CuO 4− δ sample consisted of four identical pieces with a total area of 2 × 2 cm 2 and was attached to the sample holder with a conductive Ag paint. Analysis The ZF LE-μSR data are fit [33] to a sum of two functions; P z ( t )= P LCCO + P Ag , corresponding to the signal from the fraction of muons stopping in LCCO, and the remaining fraction of muons (20–30%) stopping in the Ag mounting plate. The latter is accounted for with an exponential with a small relaxation rate of 0.02–0.04 μs −1 . The signal from the LCCO may be decomposed into a magnetic fraction f and a non-magnetic or paramagnetic fraction 1− f ; The magnetic fraction is fit to a phenomenological function consisting of three relaxation functions: (1) a weakly relaxing Kubo–Toyabe function due to nuclear moments ( σ N ≈0.05–0.1 μs −1 ). This term dominates well above the ordering temperature when the electronic moments are rapidly fluctuating but has little effect at low temperatures where the electronic moments dominate. (2) A slowly relaxing exponential, , attributed mostly to slow fluctuations in the nuclear dipolar field. (3) A term that takes into account a broad distribution of large quasi-static internal magnetic fields from the magnetism; . For simplicity, we assume the direction of the internal magnetic field is random in orientation, giving rise to the geometric 1/3 non-precessing component appearing in G mag . The parameter B represents the average internal magnetic field from the static ordering, whereas λ F characterizes the width of this field distribution. This term dominates at low temperatures in the ordered state. Since there is an interplay between B and λ F , the latter is parametrized as B = kλ F , where k is a fitted parameter. This assumes that the static width of the magnetic field distribution is proportional to the average field. In the non-magnetic fraction of the sample, only the first two terms in the relaxation function contribute. It should be noted that other fitting functions have been tested, leading to very similar results. How to cite this article: Saadaoui, H. et al . The phase diagram of electron-doped La 2− x Ce x CuO 4− δ . Nat. Commun. 6:6041 doi: 10.1038/ncomms7041 (2015).